Echo-acoustic flow dynamically modifies the cortical map of target range in bats Echolocating bats use the delay between their sonar emissions and the reflected echoes to measure target range, a crucial parameter for avoiding collisions or capturing prey. In many bat species, target range is represented as an orderly organized map of echo delay in the auditory cortex. Here we show that the map of target range in bats is dynamically modified by the continuously changing flow of acoustic information perceived during flight (‘echo-acoustic flow’). Combining dynamic acoustic stimulation in virtual space with extracellular recordings, we found that neurons in the auditory cortex of the bat Phyllostomus discolor encode echo-acoustic flow information on the geometric relation between targets and the bat’s flight trajectory, rather than echo delay per se . Specifically, the cortical representation of close-range targets is enlarged when the lateral passing distance of the target decreases. This flow-dependent enlargement of target representation may trigger adaptive behaviours such as vocal control or flight manoeuvres. In the mammalian cortex, information from peripheral sensors is typically organized as topographic representation of the sensory epithelial surfaces (‘structural maps’). For example, the primary visual, auditory and somatosensory cortices contain a retinotopic, tonotopic and somatotopic representation of the respective sensors [1] , [2] , [3] . However, cortical maps exist that are not derived by simply organizing primary inputs from the respective sensors, but contain a representation of sensory information derived by neural computation. A good example of such a computational map is the map of target range in the auditory cortex of many echolocating bats [4] , [5] , [6] , [7] . Echolocating bats use the delay between their sonar calls and the reflected echoes to measure target range, a parameter of crucial importance for avoiding collisions or capturing prey [8] , [9] . Neurons at different stages of the ascending auditory pathway have been shown to selectively encode specific call/echo delays in their response rate [10] , [11] , [12] . This echo delay selectivity has been shown to emerge in the midbrain, and is then reorganized in the dorsal auditory cortex to represent target range in an orderly organized map [13] . This map is essential for the perception of biosonar signals [14] . In natural complex environments, bats have to adapt their flight manoeuvres to the constantly changing spatial layouts. Self-motion induced echo-acoustic flow field information is readily available to tackle this challenging task. Echo-acoustic flow is the continuously changing flow of acoustic stimulation derived by echoes reflected from a target while a bat is flying. In contrast to echo delay alone, the echo-acoustic flow field provides information not only about target range but also about the geometric relationship between targets relative to the bat [15] . Both experimental and theoretical work has provided first evidence that, similar to the visual analysis of optic flow, bats perceive echo-acoustic flow [16] , [17] , [18] . During direct approach of an object, echolocation provides explicit information about the distance, as a simple linear extrapolation of the decrease in echo delay over time allows to estimate the time-to-contact. However, echo-acoustic flow field information is required to keep the lateral distance to passing objects constant, as it is often observed for bats following the edges of vegetation in commuting flight [19] . For the visual system, the cortical area MST (especially its dorsal part, MSTd) in mammals and the nucleus rotundus in birds have been shown to be important stages for the computation of visual flow field information [20] , [21] . Although there are studies on neural representation of acoustic motion in humans and animals [22] , [23] , [24] , the neural substrate underlying the analysis of acoustic flow has not been identified so far. The aim of the present study was to investigate the neural representation of echo-acoustic flow in the dorsal cortex of the bat Phyllostomus discolor . Of special interest was how the cortical map of target range, as one of the behaviourally most important parameters in echolocation, was influenced by echo-acoustic flow. We recorded the responses of cortical units to naturalistic call/echo sequences presented in virtual acoustic space via earphones. The sequences simulated the emitted sonar calls as well as the echoes a bat would perceive while passing an obstacle positioned laterally in the horizontal plane ( Fig. 1a–c ). Flight trajectories were simulated for three different lateral passing distances ( d =0.2, 0.8 and 1.4 m) and two velocities ( v =3 and 6 m s −1 ) while heading distance (distance in the direction of locomotion) and call emission rate were kept constant (4 m and 12 Hz, respectively). In the naturalistic call/echo sequences, all parameters affecting the echo-acoustic flow such as echo delay, echo reflection angle, the ratio of call amplitude and echo amplitude and echo spectral content changed in a specific manner depending on the lateral passing distance ( Fig. 1d–o ). 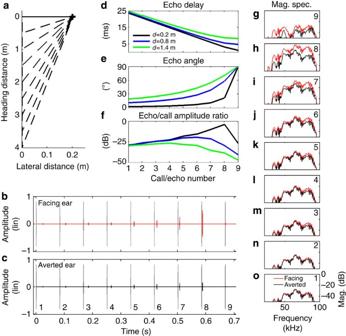Figure 1: Generation of naturalistic call/echo sequences. (a) Sketch of the spatial layout of the echo-acoustic scene. Call/echo sequences were generated for a bat starting at a heading distance of 4 m and flying lateral towards an obstacle (indicated by the bold cross at 0 m heading distance). Stippled lines indicate the echoes reflected successively from the obstacle during approach. (b,c) Naturalistic call/echo sequences were constructed by adding sonar calls (grey) and the appropriate echoes (red/black) from different positions along the flight path. The example shows the stimulus sequence presented to the ear facing the obstacle (b) and the opposite ear (c) generated for a lateral passing distance of 0.2 m and a flight velocity of 6 m s−1. Call rate was held constant at 12 Hz. Note the different progression of echo amplitudes for the sequences presented at different ears. Call/echo numbers within a sequence are indicated inc. (d–f) Progression of echo delay (d), echo angle (e) and the echo/call amplitude ratio (f) as a function of the call/echo number within a sequence for the three lateral passing distances (0.2, 0.8 and 1.4 m) used to generate naturalistic sequences. Values are presented for the ear facing the obstacle. (g–o) Magnitude spectra of the different echoes for the ear facing the obstacle (red) and the averted ear (black). Call/echo numbers within a sequence are indicated in each plot. Figure 1: Generation of naturalistic call/echo sequences. ( a ) Sketch of the spatial layout of the echo-acoustic scene. Call/echo sequences were generated for a bat starting at a heading distance of 4 m and flying lateral towards an obstacle (indicated by the bold cross at 0 m heading distance). Stippled lines indicate the echoes reflected successively from the obstacle during approach. ( b , c ) Naturalistic call/echo sequences were constructed by adding sonar calls (grey) and the appropriate echoes (red/black) from different positions along the flight path. The example shows the stimulus sequence presented to the ear facing the obstacle ( b ) and the opposite ear ( c ) generated for a lateral passing distance of 0.2 m and a flight velocity of 6 m s −1 . Call rate was held constant at 12 Hz. Note the different progression of echo amplitudes for the sequences presented at different ears. Call/echo numbers within a sequence are indicated in c . ( d – f ) Progression of echo delay ( d ), echo angle ( e ) and the echo/call amplitude ratio ( f ) as a function of the call/echo number within a sequence for the three lateral passing distances (0.2, 0.8 and 1.4 m) used to generate naturalistic sequences. Values are presented for the ear facing the obstacle. ( g – o ) Magnitude spectra of the different echoes for the ear facing the obstacle (red) and the averted ear (black). Call/echo numbers within a sequence are indicated in each plot. Full size image Our results indicate, that neurons in the dorsal auditory cortex of bats do not encode echo delay per se , as is commonly thought, but rather encode complex information about the spatial position of a target in relation to the bat’s flight trajectory. The cortical representation of close-range targets is enlarged when the lateral passing distance of the target decreases. The results demonstrate a possible neural substrate for adaptive behaviour. The enhancement of the representation of the most relevant information in a sensory map might represent a common mechanism in all vertebrates important to link perception and action in dynamically changing complex environments. Data were recorded from 145 units in the posterior dorsal auditory cortex of three bats. When tested with stimulus sequences simulated for flight speeds of v =3 m s −1 and v =6 m s −1 , 112/145 (77% ) and 111/145 (77%) units responded significantly to one or more call/echo pairs of the stimulus sequences, respectively. 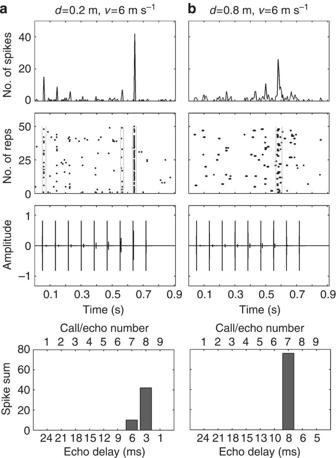Figure 2: Neurons selectively encode distinct call/echo delays within a naturalistic sequence. Reponses of units to a naturalistic sequence generated for a lateral passing distance of (a) 0.2 m and (b) 0.8 m. Flight velocity was 6 m s−1for both units. Top row: PSTH (bin width=5 ms); second row: raster plots; third row: call/echo sequence for the ear facing the obstacle and bottom row: summed spikes evoked by each call/echo pair of the stimulus sequence. In the raster plots, analysis windows for significant responses evoked by call/echo pairs are indicated by grey vertical lines. Note, that in the bottom panels spike sums are only shown for significant analysis windows. Responses evoked by the first call/echo pair of a sequence were always excluded. Different echo delays associated with the different call/echo numbers are due to the different lateral passing distances used to generate the naturalistic sequences ina,b. Figure 2 shows responses of two different cortical units to naturalistic stimulus sequences. For the unit shown in Fig. 2a , target approach was simulated for a flight velocity of 6 m s −1 and a lateral passing distance of 0.2 m. Except for the weak response evoked by the first stimulus of the sequence and an even weaker response to call/echo pair #7, only the call/echo pair with an echo delay of 3 ms (call/echo #8, bottom row) evokes a strong and significant response (stimulus-evoked neural activity is significantly stronger compared with spontaneous activity, Wilcoxon signed rank test, P >0.01, see Materials and Methods for details). Units were classified as ‘selective’ if the response evoked by one call/echo pair presented within the stimulus sequence was at least 30% stronger than the responses evoked by any other call/echo pair. The echo delay of the corresponding call/echo pair was considered as the ‘best delay’ of the unit. The unit shown in Fig. 2b is selective for a longer call/echo delay of 8 ms (call/echo #7, bottom row) when tested for a stimulus sequence simulating target approach with a lateral passing distance of 0.8 m and a flight velocity of 6 m s −1 . In total, 67% of units (75/112) and 75% of units (83/111) showed a selective response to a distinct echo delay for at least one lateral passing distance and flight velocities of 3 and 6 m s −1 , respectively. Figure 2: Neurons selectively encode distinct call/echo delays within a naturalistic sequence. Reponses of units to a naturalistic sequence generated for a lateral passing distance of ( a ) 0.2 m and ( b ) 0.8 m. Flight velocity was 6 m s −1 for both units. Top row: PSTH (bin width=5 ms); second row: raster plots; third row: call/echo sequence for the ear facing the obstacle and bottom row: summed spikes evoked by each call/echo pair of the stimulus sequence. In the raster plots, analysis windows for significant responses evoked by call/echo pairs are indicated by grey vertical lines. Note, that in the bottom panels spike sums are only shown for significant analysis windows. Responses evoked by the first call/echo pair of a sequence were always excluded. Different echo delays associated with the different call/echo numbers are due to the different lateral passing distances used to generate the naturalistic sequences in a , b . Full size image To test whether selective responses really depended on call/echo delay sensitivity, we presented sequences consisting of either only calls or only echoes. 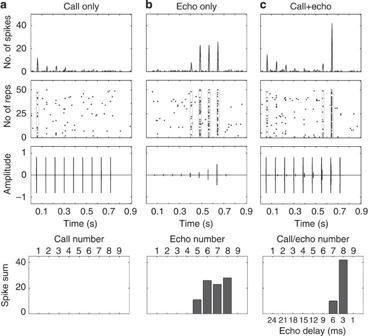Figure 3: Call/echo combination influences response selectivity. (a) Response of a cortical unit to a stimulus sequence containing only sonar calls. (b) Response of the same unit to a sequence containing only echoes. (c) Response of the same unit to a naturalistic sequence consisting of calls and echoes. Lateral passing distance was always 0.2 m, flight velocity 6 m s−1Panels are arranged as inFig. 2. In the raster plots, analysis windows for significant responses evoked by call/echo pair are indicated by grey vertical lines. Figure 3a shows a unit that only weakly responds to presentation of a call-only sequence. When an echo-only sequence was presented, the unit responded significantly and almost equally strong to echoes 6–8 ( Fig. 3b ), that is, it was not selective for a certain echo within the stimulus sequence. However, when a naturalistic sequence was presented consisting of both calls and echoes ( Fig. 3c ), the unit shows a selective response to an echo delay of 3 ms (call/echo #8, bottom row; same unit as shown in Fig. 2a ). For the large majority (177/234, 76%) of selective responses evoked by any combination of flight velocity and lateral passing distance, the selectivity depended on the presentation of naturalistic call/echo pairs in the stimulus sequences and was not observed with presentations of call-only or echo-only sequences. Figure 3: Call/echo combination influences response selectivity. ( a ) Response of a cortical unit to a stimulus sequence containing only sonar calls. ( b ) Response of the same unit to a sequence containing only echoes. ( c ) Response of the same unit to a naturalistic sequence consisting of calls and echoes. Lateral passing distance was always 0.2 m, flight velocity 6 m s −1 Panels are arranged as in Fig. 2 . In the raster plots, analysis windows for significant responses evoked by call/echo pair are indicated by grey vertical lines. Full size image Interestingly, in the unit shown in Fig. 3c , the response to call/echo pair 8 (3-ms echo delay) is stronger than the response evoked by presenting the corresponding echo only ( Fig. 3b , bottom row). In contrast to this, call/echo pairs 5–7 in the naturalistic sequence show much weaker responses than those evoked by presenting echo 5–7 only ( Fig. 3b ). This indicates that complex interactions of facilitation and suppression are underlying response selectivity for specific call/echo delays in naturalistic stimulus sequences. In a subset of 20 cortical neurons classified as ‘selective’, we tested whether selectivity also depended on the correct presentation order of call/echo pairs, an essential property of a naturalistic flow field. We presented single call/echo pairs from naturalistic sequences in random order without any temporal relationship between the different pairs. The unit in Fig. 4a shows a selective response for a delay of 12 ms (call/echo #6) when the call/echo pairs are presented in the naturalistic order. However, the same unit responds unselectively to a broad range of call/echo delays during random presentation ( Fig. 4b ). Therefore, echo delay is not the only crucial parameter underlying selectivity to certain call/echo pairs, instead the whole stimulus context of a naturalistic sequence is important. We found that 55% of neurons tested (11/20) became unselective (that is, showed a broader tuning) during random presentation, while another 30% of neurons tested (6/20) remained selective but changed their selectivity to a different best delay. Thus, in 85% of neurons tested (17/20), selective responses depended on the naturalistic presentation order. 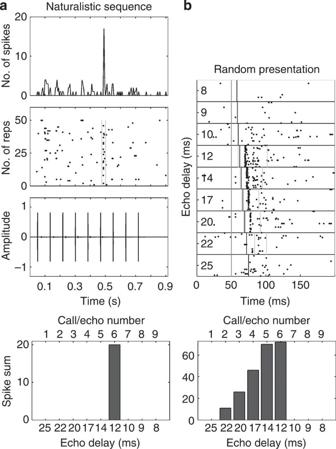Figure 4: Response selectivity depends on presentation order of call/echo pairs. (a) Response of a cortical unit to a naturalistic call/echo sequence. Lateral passing: 1.4 m, flight velocity: 6 m s−1. Panels are arranged as inFig. 2. (b) Raster plot (top) and summed spikes evoked by each call/echo pair (bottom) for random presentation (50 repetitions) of the same 9 call/echo pairs as ina. In the raster plot, call onset is indicated by the dark grey vertical dotted line. Black vertical solid lines indicate echo onset. Analysis windows for significant responses evoked by call/echo pair are indicated by grey vertical lines. Figure 4: Response selectivity depends on presentation order of call/echo pairs. ( a ) Response of a cortical unit to a naturalistic call/echo sequence. Lateral passing: 1.4 m, flight velocity: 6 m s −1 . Panels are arranged as in Fig. 2 . ( b ) Raster plot (top) and summed spikes evoked by each call/echo pair (bottom) for random presentation (50 repetitions) of the same 9 call/echo pairs as in a . In the raster plot, call onset is indicated by the dark grey vertical dotted line. Black vertical solid lines indicate echo onset. Analysis windows for significant responses evoked by call/echo pair are indicated by grey vertical lines. Full size image We analysed the representation of best echo delay on the cortical surface of P. discolor as a function of the lateral passing distance between the obstacles and the simulated flight trajectories. The best delay of a unit was derived for units that responded selectively to a distinct call/echo pair within a stimulus sequence. As this method focuses only on a single point (that is, call echo pair) within the whole stimulus sequence, an additional analysis method was used that provided a broader, more ‘global’ evaluation of the complete response evoked by the naturalistic stimulus sequence. For this purpose, the response of a unit was arranged as a peristimulus time histogram (PSTH, 1 ms bin width) and convolved with a Gaussian window. The peak value of the PSTH after convolution was determined and the theoretical echo delay time at this point was calculated and considered as the ‘best delay’ of this cortical unit. 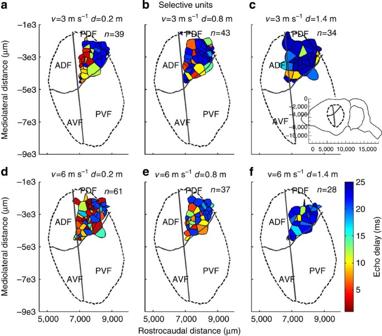Figure 5: Cortical representation of best echo delay of selective units changes with lateral object distance. Voronoi–tessellation maps of best delay of selective units projected onto the flattened surface of the AC for three different lateral passing distances (0.2, 0.8 and 1.4 m) for a fight speed of 3 m s−1(a–c) and a flight speed of 6 m s−1(d–f). Polygons mark cortical recording sites for particular best delays. The size of the polygons reflects the spatial density of recording sites on the cortical surface. The borders of the AC are indicated by dotted lines and the borders of the auditory cortical subfields are indicated by solid lines. ADF, anterior dorsal field; AVF, anterior ventral field; PVF, posterior ventral field. Outlines of cortical fields are shown according to ref.57. The insert incshows the outlines of the AC on a schematic theP. discolorbrain. Figure 5 shows tessellation maps of the best delay of units classified as ‘selective’ projected on the cortical surface of P. discolor . Most recordings were derived from the posterior dorsal field (PDF), with only few outliers located close to the borders of the PDF in adjacent fields. For stimulus sequences simulated for both flight velocities (3 and 6 m s −1 ) the tessellation maps show that the representation of best delay clearly changes with the lateral passing distance of the simulated flight path. For a lateral passing distance of 0.2 m, short delays in the range up to ~12 ms are represented in the frontal half of the PDF ( Fig. 5a,d ). However, the representation of short delays is progressively reduced when the lateral passing distance increases ( Fig. 5b,c,e,f ). From Fig. 5c,f it can be clearly seen that for a passing distance of 1.4 m (range of echo delays: 8–25 ms, see also Fig. 1d ) areas of the cortical surface in the frontal part of the PDF that represented short delays for a passing distance of 0.2 m (range of echo delays: 1 and 24 ms) now represent longer delays. The representation of best delays in the caudal part of the PDF, however, shows no systematic modifications in dependency on lateral passing distance. Figure 5: Cortical representation of best echo delay of selective units changes with lateral object distance. Voronoi–tessellation maps of best delay of selective units projected onto the flattened surface of the AC for three different lateral passing distances (0.2, 0.8 and 1.4 m) for a fight speed of 3 m s −1 ( a – c ) and a flight speed of 6 m s −1 ( d – f ). Polygons mark cortical recording sites for particular best delays. The size of the polygons reflects the spatial density of recording sites on the cortical surface. The borders of the AC are indicated by dotted lines and the borders of the auditory cortical subfields are indicated by solid lines. ADF, anterior dorsal field; AVF, anterior ventral field; PVF, posterior ventral field. Outlines of cortical fields are shown according to ref. 57 . The insert in c shows the outlines of the AC on a schematic the P. discolor brain. Full size image The same trend can be seen for the tessellation maps of best delay derived by the Gaussian window method shown in Fig. 6 . This is especially important, as the higher number of data points available with this method confirms that the lateral passing distance-dependent changes in cortical representation of best delay are due to a robust effect. It is important to note that the range of best delays of units in the frontal part of the PDF is not restricted to the range below 8 ms, but includes also best delays around 10 ms or even somewhat higher. The change towards a representation of longer best delays in the frontal part of the PDF can therefore not simply be attributed to the different range of echo delays contained in the different stimulus sequences. 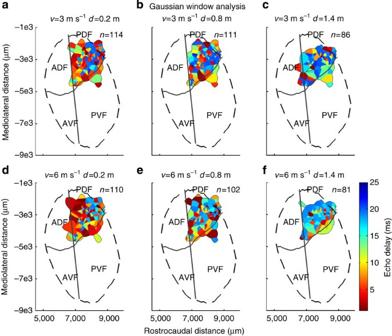Figure 6: Cortical representation of best echo delay obtained from smoothed responses changes with lateral object distance. Voronoi–tessellation maps of best delay derived by convolution of PSTHs of cortical units with a Gaussian window. Maps for three different lateral passing distances (0.2, 0.8 and 1.4 m) for a fight speed of 3 m s−1(a–c) and a flight speed of 6 m s−1(d–f) are projected onto the flattened surface of the AC. Abbreviation of cortical field names same as inFig. 5. Figure 6: Cortical representation of best echo delay obtained from smoothed responses changes with lateral object distance. Voronoi–tessellation maps of best delay derived by convolution of PSTHs of cortical units with a Gaussian window. Maps for three different lateral passing distances (0.2, 0.8 and 1.4 m) for a fight speed of 3 m s −1 ( a – c ) and a flight speed of 6 m s −1 ( d – f ) are projected onto the flattened surface of the AC. Abbreviation of cortical field names same as in Fig. 5 . Full size image The higher number of data points also allowed for a more detailed analysis of the observed changes in the cortical delay map. In principle, the observed systematic, lateral passing distance-dependent shift in the cortical delay map can be due to three different response pattern changes at the level of individual cortical units: (1) the unit responds to both short and long lateral passing distances equally strong but shows a shift in the best delay, (2) the unit responds only to short lateral passing distances at short delays and becomes silent to long lateral passing distances or (3) the unit does not respond to short lateral passing distances but responds to long lateral passing distances at long delays. All of these three response types were observed in cortical units of P. discolor . Complete data sets with recordings for all three lateral passing distances and both flight velocities were analysed for 114 units. 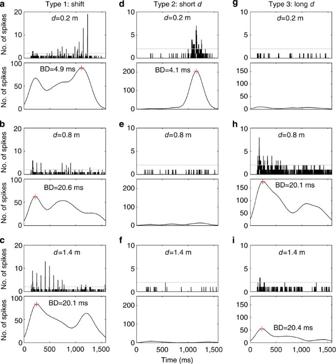Figure 7: Lateral passing distance induces different responses in cortical units. (a–c) PSTH (1 ms bin width, top) and response profile after convolution with a Gaussian window (bottom) for a cortical unit that increases its best delay (BD, indicated by a red cross) when lateral passing distance is increased from 0.2 m (a) to 0.8 (b) and 1.4 m (c). (d–f) Response of a cortical unit that only responds to short lateral passing distances and (g–i) a unit that only responds to medium and long lateral passing distances. Flight velocity was always 3 m s−1. The horizontal grey line in the PSTHs indicates the level of three spikes per bin that was used as response threshold required for convolution with the Gaussian window. Shortest and longest echo delay presented in the stimulus sequences were 1 and 24, 5 and 24 and 8 and 25 ms for lateral passing distance of 0.2, 0.8 and 1.4 m, respectively. Figure 7 shows examples from units tested with call/echo sequences simulated for flight velocities of v =3 m s −1 . In the unit shown in Fig. 7a–c , the best response shifts from short delay to long delay when the lateral passing distance is increased from 0.2 to 1.4 m, although the response to 0.8 m passing distance is somewhat reduced. In total, 49 of 114 units (43%) displayed this general type of response pattern. The unit in Fig. 7d–f responds only to a short delay when the lateral passing distance is 0.2 m but shows no strong response to any delay at all when the lateral passing distance is increased. This type of response pattern was observed in 14/114 units (12%). An opposite response pattern is shown in Fig. 7g–i : the unit shows its strongest response peak for long delays when the lateral passing distance is 0.8 m and also clearly responds to long delays when the lateral passing distance is 1.4 m; but it does not respond strongly for a lateral passing distance of 0.2 m (8/114; 7%). For flight velocities of 6 m s −1 , the corresponding frequency of occurrence of the three response types were 42/114 (37%), 14/114 (12%) and 9/114 (8%). Figure 7: Lateral passing distance induces different responses in cortical units. ( a – c ) PSTH (1 ms bin width, top) and response profile after convolution with a Gaussian window (bottom) for a cortical unit that increases its best delay (BD, indicated by a red cross) when lateral passing distance is increased from 0.2 m ( a ) to 0.8 ( b ) and 1.4 m ( c ). ( d – f ) Response of a cortical unit that only responds to short lateral passing distances and ( g – i ) a unit that only responds to medium and long lateral passing distances. Flight velocity was always 3 m s −1 . The horizontal grey line in the PSTHs indicates the level of three spikes per bin that was used as response threshold required for convolution with the Gaussian window. Shortest and longest echo delay presented in the stimulus sequences were 1 and 24, 5 and 24 and 8 and 25 ms for lateral passing distance of 0.2, 0.8 and 1.4 m, respectively. Full size image Thus, although response strength could vary non-monotonically, about 60% of units changed their response preference systematically in a way that contributes to the systematic shift of the cortical map of delay. In the remaining units, response changes were absent or completely unsystematic. We quantified the extent of changes in the cortical representation by calculating the percentage of neurons responding to echo delays of 12 ms or shorter (representing target range of <=2 m) for each lateral passing distance and the two different flight velocities. Please note, that echo delays shorter than 12 ms are well represented in all stimulus sequences ( Fig. 1d ). 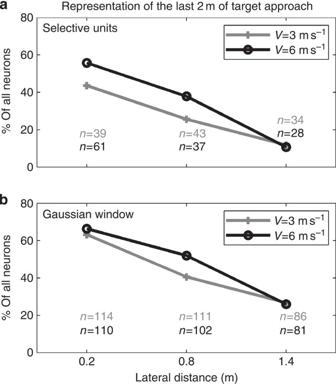Figure 8: Cortical representation of the last two metres of target approach. (a) Percentage of all cortical neurons responding to echo delays of 12 ms or shorter (representing target range of <=2 m) for each lateral passing distance and the two different flight velocities as derived for delay selective units and (b) derived from Gaussian window analysis. Figure 8 shows the result of this quantification for the best delays of selective units ( Fig. 8a ) and the delays derived with the Gaussian-window method ( Fig. 8b ). For both methods, the percentage of neurons selectively responding to short best delay (representing target ranges up to 2 m) increases with decreasing lateral object distance ( Fig. 8a,b ). Most importantly, the increase is more pronounced when the flight trajectory is simulated for higher flight speeds. Figure 8: Cortical representation of the last two metres of target approach. ( a ) Percentage of all cortical neurons responding to echo delays of 12 ms or shorter (representing target range of <=2 m) for each lateral passing distance and the two different flight velocities as derived for delay selective units and ( b ) derived from Gaussian window analysis. Full size image To summarize, the cortical representation of best delay/target range changes depends on the lateral passing distance and flight velocity: short delays are more strongly represented for short lateral distances and higher velocity. The cortical map of target range appears not to be ‘fixed’ but is to be adjustable according to acoustic flow information. Echo delay per se is not the most important encoded parameter, but encoding depends also on additional parameters. In the present study, we investigated the influence of echo-acoustic flow information on the cortical computational map of target range in bats. The results show that the map of target range is modified by echo-acoustic flow in a situation-specific manner. With decreasing lateral target distance in simulated flight trajectories, the representation of close targets, that is, short echo delays, is increased. The effect is stronger when flight trajectories are simulated at higher flight speeds. The results show that a computational cortical map can be dynamically adapted depending on situation-specific sensory input, thereby enhancing the representation of the most relevant information. Our study uses naturalistic call/echo sequences. The echoes in these sequences were generated as spatially dependent reflections of a single target. At first glance, this seems to be a fairly artificial spatial layout, as one would expect that in most natural environments, a single call would evoke a multitude of echoes reflected by a multitude of objects along the flight path of the bat. However, it was shown in behavioural experiments with free-flying bats that bats focus on single targets along their flight path by carefully steering their sonar beam to sequentially scan all targets, but ensonifying only one confined target or point in space at a time [25] . The number of echoes evoked by single calls is thereby reduced. Our stimulus sequence can therefore be considered representative for the spatial sonar information gained by a flying bat. The temporal structure of the emitted calls in flight, however, might be different in a naturalistic situation. Flying bats typically emit their sonar calls in temporally structured strobe groups and emission rate is increased when a target is directly approached [26] . These temporal features were not included in our stimulus sequences to avoid an excess of parameters that might influence the neuronal response. Strobe groups are assumed to play a role in the segregation of complex echo-acoustic scenes [26] . The scope of the present experiments was to investigate the influence of acoustic flow on the cortical representation of target range, that is., call echo delay. The implementation of strobe groups in the experimental design seemed therefore not compelling but should of course be taken into account in more specialized experiments on auditory scene analysis. Theoretical analyses showed that echo-acoustic flow provides multiple cues that can be used by bats for target localization during translational movements within a plane [16] , [17] , [18] . In addition to changes in Doppler frequency that are most important for CF bats and were therefore not considered in our stimulus paradigm, proportional changes in echo intensity, echo delay or echo reflection angle are considered to be potential cues that could be perceived by bats. So far, the results from psychophysical studies were inconclusive regarding the relative importance of these cues [16] . The electrophysiological results of our study suggest that echo delay might by the most important parameter: response selectivity for a certain target distance during target approach was mainly observed for naturalistic stimulus sequences containing both calls and echoes. However, the detailed weighting of the other cues (echo intensity and reflection angle) remains to be quantified in future studies. Focal electrical stimulation of auditory cortical neurons in bats is known to evoke reorganization of subcortical and cortical areas [27] , [28] , [29] . In detail, stimulation of distinct positions in the cortical map of target range evokes centrifugal shifts in best echo delay (that is, away from the best delay of the stimulated site) of neurons in close-by locations [30] . In other mammals, task-dependant plasticity in the auditory cortex has been shown for tone amplitude [31] , tone frequency [32] temporal sound modulation [33] and spectrotemporal tuning properties of cortical neurons [34] , [35] , [36] , [37] . Common to all these plasticity effects is, however, that they typically occur on a long or medium time scale of at least minutes. In contrast, the changes in the cortical representation of target range in our study were observed ad hoc , and did not rely on excess stimulation. The changes are thus not likely to be based on the same mechanisms underlying classical plasticity, for example, modifications of synaptic strength or structural changes such as formation or morphological remodelling of cortical synapses [38] . It is more likely that the changes occur on a computational basis. Support for this thesis comes from a recent study [7] , in which it was shown that the map of target range in several bat species has a multiparametric nature and is therefore not precise, but blurry. In detail, the delay-tuning of auditory cortical neurons depended on which spike output parameters (for example,, echo delay at maximum response or echo delay at response threshold) was used to characterize the responses. In addition, several studies showed that delay-tuning of cortical and subcortical neurons is influenced by several parameters such as call/echo level ratio [39] , [40] and spatial position [41] . The single pulse-echo pairs from the stimulus sequences used in our study show a variation of all these parameters during virtual target approach and in relation to the lateral passing distance ( Fig. 1 ). Interestingly, the cortical activation pattern shown by Hechavarria [7] for different statically presented combinations of echo level and echo delay strongly resembles the activation patterns evoked by echo-acoustic flow information: the map of target range is blurry for most echo level and echo delay combinations except for those only activating the most caudal part of the map representing long delay/target distance. In our study, the part of the cortical map of target range representing short and medium target distances (that is, the frontal and middle parts of the PDF) is also prone to the largest flow-dependent changes ( Figs 5 and 6 ). The variable, multiparametric nature of the map of target range in bats seems to be a general feature of cortical maps and has also been observed in structural maps in the primary auditory cortex of mammals [42] , [43] as well as in other computational maps such as the auditory space map in the tectum of the barn owl [44] . Furthermore, ad hoc changes in spatial representations have also been shown to occur across different sensory modalities, for example, auditory spatial receptive fields in the superior colliculus of primates were influenced by gaze direction [45] . Apart from the capture of prey on the wing, obstacle avoidance is one of the major tasks bats perform on the basis of echolocation. In addition, while commuting between roosts and feeding grounds, bats often fly closely along natural structures like edges of canopy [19] . The dynamic nature of the echo-acoustic information a bat perceives during flight imposes a major challenge to both the sensory and motor systems: bats have to dynamically adjust their sonar emission and flight manoeuvres according to the required task [46] . The echo-acoustic flow-dependent changes of echo delay representation on the cortical surface observed in the present study may represent a neural substrate to optimally accomplish all these tasks: (1) The representation of close-by targets (that is, short echo delays) increases when the bat decreases the lateral passing distance relative to a target. This makes sense as the risk of undesired collision increases under this condition. The bat would need more accurate information about target distance and position. Both types of information can be derived from acoustic flow information [17] and would therefore be strongly represented on the cortical surface. In this respect, it is important to notice that the response of cortical units depends not just on single pulse-echo pairs, but is influenced by the complete stimulus sequence ( Fig. 4 ). Therefore, the cortical responses also represent information about the recent flight path and thus also about the geometry of the obstacle arrangement. (2) The increase of the cortical area dedicated to the representation of close-by targets was stronger for higher flight velocities. Typically, a stronger representation of a sensory parameter in a map results in faster reaction times and increased action precision [47] . Hence, this mechanism would enable the bat to react faster and initiate adequate flight manoeuvres as would be required due to higher flight velocities. The increasing representation of a certain target on the cortical surface could be used to trigger different kinds of motor behaviour including vocal control of sonar signal duration and timing and control of flight manoeuvres. Theoretically, this could be implemented in the neural circuitry as a simple threshold mechanism, by which a specific motor pattern is initiated whenever cortical activity in the map of target range exceeds a critical amount. Such a mechanism would be somewhat similar to what has been described for visual looming [21] : neurons in the nucleus rotundus of birds start to fire if the increase of the visual angle subtended on the retina by an approaching object exceeds a certain amount within a certain time. Unlike the visual system, in the auditory system the peripheral sensors do not have a two-dimensional layout. Therefore, a threshold mechanism of this kind would necessarily have to be implemented centrally, that is, as the dynamical increase of activity in a cortical map. As an additional interpretation, the findings of our study may also hint towards a neural substrate that combines information about distance and angular position of a target. In the visual system, the inferior parietal cortex is an important structure to compute the absolute metrics of a target and its position in egocentric coordinates [48] . However, the best delay of a cortical unit does not simply depend on a static combination of target distance and target angle. Our results show that dynamic stimulus aspects are important: the order of pulse/echo stimuli presentation has a strong effect on the best delay of a unit ( Fig. 4 ). The fact that the cortical representation of the last two metres of target approach is depending on flight velocity ( Fig. 8 ) in addition emphasizes the notion that dynamic spatiotemporal acoustic input is an important determinant for the responses of cortical neurons in the bat P. discolor . In conclusion, the present results demonstrate a neural substrate for task-specific adaptive behaviour. The cortical map of target range is dynamically modified according to the requirements of the actual situation by increasing the cortical representation of the most relevant information. Surgery All experiments complied with the principles of laboratory animal care and were conducted under the regulations of the current version of the German Law on Animal Protection (approval 55.2-1-54-2531-128-08 Regierung von Oberbayern). All bats ( P. discolor; two adult females and one adult male) originated from a breeding colony in the Department Biology II of the Ludwig-Maximilians-University in Munich. For experiments, animals were kept separated from other bats under semi-natural conditions (12 h day per 12 h night cycle, 65–70% relative humidity, 28 °C) with free access to food and water. The principle surgical procedure has been described in detail elsewhere [5] and will be mentioned here in the following only in brief: The bats were anesthetized using a combination of medetomidine (Domitor, Novartis, Mississauga, Canada), midazolam (Dormicum, Hoffmann-La Roche, Mississauga, Canada) and fentanyl (Fentanyl-Janssen, Janssen-Cilag, Neuss, Germany; 0.4, 4 and 0.04 μg per gram bodyweight, respectively). The skin overlying the skull was opened along the midline and the skull surface was freed from tissue. A small metal tube was fixed to the skull using a microglass composite to fixate the animal to a stereotaxic device, and the accurate skull position in stereotaxic coordinates was determined as described in detail elsewhere [49] . In brief, the alignment of the animal’s skull and brain within the stereotaxic coordinate system was measured by scanning characteristic profile lines of the skull in the parasagittal and frontal plane. These profiles were then fitted to a standardized skull profile in a standardized coordinate system. To alleviate postoperative pain, an analgesic (0.2 mg kg −1 bodyweight Meloxicam, Metacam, Boehringer-Ingelheim, Ingelheim, Germany) was administered after the surgery. Stimulus generation and electrophysiological recordings Experiments were conducted in a sound-attenuated chamber. Extracellular recordings were made with conventional glass insulated tungsten electrodes (1–2 MOhm impedance, Alpha Omega GmbH, Ubstadt-Weiher, Germany) in anesthetized bats (medetomidine, midazolam and fentanyl (0.4, 4 and 0.04 μg per gram bodyweight, respectively)). During recording, anaesthesia was maintained by injecting half of the initial dose of the anaesthetic every 2 h. Note that responses recorded from cortical units under this anaesthesia regime reflected the behavioural performance of P. discolor well [50] . Recording sessions could last up to 4 h per day and were repeated on 4 days a week. Electrode penetrations in the AC were run oblique to the brain surface with different mediolateral and rostrocaudal angles. Because it was not always possible to clearly discriminate the activity of a single neuron, the term ‘unit’ will be used in the following to describe the collective activity of one to three neurons recorded at a recording site. Naturalistic call/echo sequences to simulate echo-acoustic flow were generated as follows: Flight trajectories were calculated for a bat flying laterally towards an obstacle, and the positions along the flight path in the horizontal plane were determined at which reflected echoes would reach the bat ( Fig. 1a ). The obstacle was assumed to be a perfect reflector (target strength=0 dB). Trajectories were calculated for three different lateral passing distances ( d =0.2, 0.8 and 1.4 m) and two velocities ( v =3 and 6 m s −1 ). The initial heading distance in flight direction was always 4 m and the call rate was assumed to be constant at 12 Hz, which is well in the range of call rates observed for P. discolor in flight [51] . Due to the constant rate of call emission, a slower flight speed of 3 m s −1 resulted in higher spatial sampling density. P. discolor emits its sonar calls through the nostrils, the prominent nose-leaf imposing a high degree of directionality on the calls [52] . To generate call/echo sequences, a typical call (duration about 1.2 ms, main energy between 40 and 90 kHz) was recorded from a frontal position at 0° azimuth and elevation (the call was supplied by courtesy of C. Geberl, Department Biology II, LMU Munich). All directional information was removed from this call by deconvolution with the impulse response from this position derived from the transfer function of call emission [52] . This was done because (1) it can be assumed that the bat’s cochlea is stimulated by its own call with no special spatial directionality due to bone conductance, (2) the directionality of hearing does not provide much information for the acoustic near-field and (3) the calls were also used to generate echoes reflected from different spatial directions along the simulated qflight path (see below), which requires consideration of the corresponding directionalities of emission. Therefore, an echolocation call of P. discolor containing no directionality was convolved with a left and right ear pair of the head-related transfer function and the transfer function of call/emission of P. discolor [52] , [53] corresponding to the angular direction of echo reflection for each position along the flight path. The resulting echoes included all relevant spatial cues such as ITDs, frequency-dependent IID and spectral profile. Calls (with no directionality) and echoes were then combined with the appropriate delay (between 1 and 25 ms) to generate the final stimulus sequence for all passing distances and flight velocities ( Fig. 1b,c ). Before this, calls were attenuated by 26 dB, as this is the typical level of self-stimulation relative to the sound pressure level (SPL) of call emission [54] . In the final sequences, echo-acoustically important parameters such as echo delay, echo reflection angle, the ratio of call amplitude and echo amplitude and echo spectral content changed in a specific manner depending on the lateral passing distance ( Fig. 1d–o ). Shortest and longest echo delay presented in the stimulus sequences were 1 and 24, 5 and 24 and 8 and 25 ms for lateral passing distance of 0.2, 0.8 and 1.4 m, respectively. The final echo sequences had durations of 1.34 and 0.67 s for flight velocities of 3 and 6 m s −1 , respectively. Sequences were presented binaurally, with the echoes reflected to the ear directly facing the reflector being presented to the contralateral ear with respect to the recording site. The presentation level was typically adjusted such that the loudest (contralateral) echo was presented with 70–80 dB SPL. As maximum echo amplitude differences covered a range of about 40 dB over all sequences, this ensured that faint echoes were above threshold for most units. The calls included in the stimulus sequences had the same SPL in both ears remaining constant during the sequence. Each stimulus sequence was preceded by a 50 ms silent period to determine the level of spontaneous activity (see below). In addition to the naturalistic stimulus sequences containing calls and echoes, sequences were presented that either contained only calls or only echoes. This was done to test whether responses really specifically depended on naturalistic call/echo presentation. For a subset of units, call/echo pairs derived from the different naturalistic sequences were also presented in randomized order with a repetition rate of 1.3 Hz. This allowed to test whether responses to single call/echo pairs within a sequence depended on the naturalistic presentation order and timing or were independent of acoustic flow. All stimulus sequences were DA converted (RX6, Tucker Davis Technologies, Gainesville, FL, sampling rate 260 kHz) and presented binaurally to the bats via custom made earphones with a flat frequency response ±3 dB between 10 and 100 kHz [55] . Stimulus sequences were presented with 50 repetitions and 750-ms pause after the last stimulus of a sequence and the next presentation. Action potentials were recorded using an AD converter (RA16, RX5, (TDT) sampling rate 25 kHz, band pass filter 300–3,000 Hz) and Brainware (TDT). To search for acoustically driven neural activity pairs of typical echolocation calls of P. discolor were used (downward modulated, multiharmonic, with main energy between 40 and 90 kHz and duration about 1.2 ms). The delay and amplitude ratio between both calls could be varied (DA converter: RX6 (TDT, sampling rate 260 kHz), attenuator: PA5 (TDT)). Search stimuli were presented with a repetition rate of 1.3 Hz. After the completion of an experiment, electrolytic lesions were made to the brain to reconstruct the position of recording sites from subsequent histological processing in standardized stereotaxic coordinates of a brain atlas of P. discolor (A. Nixdorf, T. Fenzl, B. Schwellnus, unpublished). Animals were then euthanized by an intraperitoneally applied lethal dose of pentobarbital (0.16 mg g −1 bodyweight) and subsequently transcardially perfused. Data analysis Data were analysed with MATLAB (MathWorks). Spike responses evoked by the different stimulus sequences were arranged as PSTHs, (5 ms bin width) and raster -plots. To determine significant responses to the different call/echo stimuli within a sequence, the raster plots were analysed using a sliding window to determine the individual response durations with a sequence [56] . The analysis windows were set automatically by moving a 10-ms window in 1-ms steps over the time course of recorded activity. The first point at which two successive windows led to significant differences (Wilcoxon signed rank test, P >0.01) in neuronal activity compared with the first 10 ms window (spontaneous activity recorded before the stimulation) was taken as the start of each analysis window. The end of each analysis window was set to the last position of two successive windows that differed significantly from spontaneous activity. For each stimulus sequence, spikes occurring in each analysis window were summed. Responses evoked by the first call/echo pair in a sequence were excluded from further analysis. This is justified as the presentation of the first stimulus of a sequence is not considered part of a dynamic scene and thus often evoked a response simply due to the onset of acoustic stimulation. Units were classified as ‘selective’ if the response evoked by one call/echo pair presented within the stimulus sequence was at least 30% stronger than the responses evoked by any other call/echo pair. The echo delay of the corresponding call/echo pair was considered as the ‘best delay’ of the unit. The method of setting analysis windows allowed the analysis of interactions like facilitation or inhibition between calls and echoes within a stimulus sequence. However, the above-mentioned criterion for response selectivity is very strict and focuses only on a certain point within the whole stimulus sequence. Therefore, an additional analysis method was used that allowed a broad, more ‘global’ evaluation of the complete response evoked by the naturalistic stimulus sequence. For this purpose, the response over all 50 repetitions was arranged as a PSTH (1 ms bin width) and convolved with a Gaussian window. Depending on the flight speed for which the stimulus sequence was generated (3 and 6 m s −1 ), the Gaussian window had a length of 500 or 250 ms, respectively. Therefore, for both sequences, the window length includes about one third of the stimulus length and covers the same spatial range of echo angles, but integrates over different numbers of echoes. Responses to the first pulse/echo pair were excluded from analysis by setting the PSTH to zero for the time period before occurrence of the second pulse of each sequence. The peak value of the PSTH after convolution with the Gaussian window was determined and the theoretical echo delay time at this point was calculated and considered as the ‘best delay’ of a cortical unit. PSTHs that did not contain more than three spikes in at least one bin were discarded from analysis to avoid unspecific response peaks after convolution. It is inevitable that peak values after convolution were assigned to pulse-echo delays that were not actually tested. However, as the spacing of the delay steps in the sequences is quite homogeneous and in no case larger than 3 ms, the Gaussian window convolution should reliably reflect the temporal envelope of the PSTH also for the pulse-echo delays not included in the stimulus sequences. Distribution of best delay on the cortical surface is represented with the help of the Voronoi–tessellation procedure in two dimensions implemented with Matlab. In detail, recording sites for units with a certain best delay are connected with all neighbouring recording sites. Cells characterizing the value of a particular parameter around recording sites are constructed as polygons whose sides pass equidistantly between recording sites and intersect the connection lines perpendicularly. How to cite this article : Bartenstein, S. K. et al . Echo-acoustic flow dynamically modifies the cortical map of target range in bats. Nat. Commun. 5:4668 doi: 10.1038/ncomms5668 (2014).